The phospholipase D1 pathway modulates macroautophagy Although macroautophagy is known to be an essential degradative process whereby autophagosomes mediate the engulfment and delivery of cytoplasmic components into lysosomes, the lipid changes underlying autophagosomal membrane dynamics are undetermined. Here, we show that phospholipase D1 (PLD1), which is primarily associated with the endosomal system, partially relocalizes to the outer membrane of autophagosome-like structures upon nutrient starvation. The localization of PLD1, as well as the starvation-induced increase in PLD activity, are altered by wortmannin, a phosphatidylinositol 3-kinase inhibitor, suggesting PLD1 may act downstream of Vps34. Pharmacological inhibition of PLD and genetic ablation of PLD1 in mouse cells decreased the starvation-induced expansion of LC3-positive compartments, consistent with a role of PLD1 in the regulation of autophagy. Furthermore, inhibition of PLD results in higher levels of Tau and p62 aggregates in organotypic brain slices. Our in vitro and in vivo findings establish a role for PLD1 in autophagy. Macroautophagy (hereafter referred to as autophagy) is an essential cellular process that mediates the lysosomal degradation of defective organelles and long-lived proteins, as well as protein aggregates [1] , [2] . Consistent with a primary role in cell homeostasis, perturbation of this pathway has been linked to disease [3] , [4] , [5] . Macroautophagy is the best-characterized autophagy pathway and involves the “bulk” degradation of portions of the cytoplasm through sequestration by a growing limiting membrane that seals to form a double membrane compartment referred to as the autophagosome (AP). The biogenesis of APs involves the recruitment of ubiquitin-like protein LC3 (and its related family members) onto membranes and covalent attachment of phosphatidylethanolamine to its cleaved COOH terminus through a conjugation system analogous to the one that mediates ubiquitination [1] , [2] , [3] , [6] . Once formed, APs can fuse with endosomes, thus generating amphisomes, which, in turn, fuse with lysosomes, so that contents can be degraded [1] , [2] , [3] , [7] , [8] . Although autophagy involves a drastic biogenesis and/or remodelling of intracellular membranous organelles, the role lipids and lipid enzymes have in this process is poorly understood. A key event in autophagy is the production of phosphatidylinositol 3-phosphate (PI(3)P) by the class III PI-3 kinase Vps34, which controls the biogenesis and maturation of APs through a variety of complexes [4] , [8] , [9] , [10] , [11] , [12] . PI(3)P also has a fundamental role in endosomal trafficking [13] ; thus, a key question is how a single lipid can achieve such critical and diverse functions in cells. A partial answer lies in the nature of PI(3)P effectors resident in endosomal or autophagosomal membranes that confer local and specific signalling properties. Indeed, several PI(3)P-binding proteins have been described, and most of them contain either a FYVE or a PX domain [13] and have been localized to early endosomes where PI(3)P is concentrated [13] . PI(3)P effectors specific to autophagy, such as DFCP1 and mammalian orthologues of Atg18 (that is, WIPI), have also been reported [14] , [15] , but do not wholly account for the complexity of Vps34 actions in autophagy. In a limited screen of lipid enzymes potentially implicated in starvation-induced autophagy either through direct effects on PI(3)P (for example, myotubularins) or as PI(3)P effectors (for example, PX domain-containing enzymes), we identified PX domain-containing enzyme phospholipase D1 (PLD1) as a potential player in autophagy. PLD1 hydrolyses phosphatidylcholine (PC) to produce the bioactive lipid phosphatidic acid (PA), which has been reported to facilitate budding from the Golgi complex, exocytosis, endocytosis and phagocytosis, as well as modulating many key signalling cascades including the mTOR pathway [16] , [17] , [18] , [19] . In yeast, the sole PLD orthologue, Spo14, is dispensable for cells in their vegetative state, but is essential for sporulation-associated prospore membrane biogenesis [20] , a process that is reminiscent of AP formation. Recent work has also pointed to a key role of Spo14 from Pichia pastoris in the unconventional secretion of Acb1 [21] . Collectively, these studies implicate PLD and its product PA in various aspects of membrane traffic, including membrane fusion. In this study, we explore the role of PLD1 in the autophagy process in mammalian cells. Our results from in vitro and in vivo experiments identify PLD1 as an important regulator of AP membrane dynamics during starvation-induced autophagy and suggest a role for this lipid enzyme in the maturation step downstream of PI-3 kinase Vps34. Additionally, our data point to a role for PLD1 in the regulation of protein aggregate clearance, with important implications for disorders associated with proteinopathies. PLD1 partially co-localizes with LC3 during starvation Nutrient deprivation, which induces autophagy, was used as a model to assess changes in the subcellular localization of PLD1 and PLD2 in both HeLa and CHO cells and their relationship with the AP marker, LC3. As reliable antibodies for the detection of endogenous PLD isoforms are unavailable, green fluorescent protein (GFP)- or haemagglutinin (HA)-tagged versions of PLD1 and PLD2 were expressed and imaged using confocal microscopy. GFP–PLD1, but not GFP–PLD2, was found to partially co-localize with mRFP–LC3 upon nutrient deprivation ( Supplementary Fig. S1a,b ). These results, which were obtained from a larger screen of lipid enzymes potentially co-localizing with LC3, prompted us to further characterize the subcellular localization of PLD1, its relationship with endogenous LC3 and its implication in autophagy. In normal medium and in partial agreement with previous reports [17] , [18] , HA–PLD1 is predominantly found in the endolysosomal system, with a significant pool co-localizing with Lamp1 (late endosomes/lysosomes) and to a lesser extent with EEA1 (early endosomes) and Vps35 (retromer-positive endosomes; Supplementary Fig. S2 ). Traces of HA–PLD1 were also found at the plasma membrane, but not on the Golgi complex (giantin, Supplementary Fig. S2 ). Immuno-electron microscopy (EM) using anti-GFP antibodies showed the enrichment of GFP–PLD1 on tubular endosome-like structures in the presence of normal medium ( Supplementary Fig. S3 ). Importantly, although endogenous LC3 was hardly detectable in normal medium, clear LC3-positive puncta appeared as a result of nutrient deprivation ( Fig. 1a ). Co-localization of LC3-positive structures with HA–PLD1 was obvious after 1 h, but was further enhanced after 2 h of nutrient deprivation, as LC3 puncta became larger and more numerous ( Fig. 1a ). 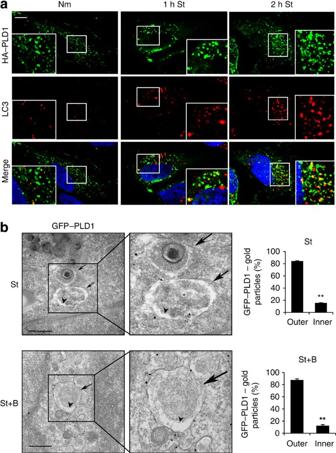Figure 1: PLD1 partially co-localizes with endogenous LC3 and is found on the outer membrane of autophagosome-related structures. (a) Confocal analysis of the subcellular localization of HA–PLD1 (green) and endogenous LC3 (red) in HeLa cells in normal medium and under nutrient deprivation conditions. Left panels: normal medium condition (Nm); middle panels: 1 h with nutrient-deprived medium (1 h St); right panels: 2 h with nutrient-deprived medium (2 h St). Insets denote high magnification of the selected area. Scale bar, 5 μm. (b) Immuno-gold EM micrographs of HeLa cells transfected with GFP–PLD1 and subjected to 1 h of nutrient deprivation in the presence (St+B) or absence (St) of bafilomycin (50 nM). Insets denote high magnification of the selected area. Scale bar, 500 nm. Right panel: Histogram showing morphometric analysis of the relative distribution of GFP–PLD1-positive gold particles on the outer (arrows) and inner (arrowheads) membranes of the autophagosomal-like structures. Values denote means±s.e.m. (n=14). **P<0.01. Figure 1: PLD1 partially co-localizes with endogenous LC3 and is found on the outer membrane of autophagosome-related structures. ( a ) Confocal analysis of the subcellular localization of HA–PLD1 (green) and endogenous LC3 (red) in HeLa cells in normal medium and under nutrient deprivation conditions. Left panels: normal medium condition (Nm); middle panels: 1 h with nutrient-deprived medium (1 h St); right panels: 2 h with nutrient-deprived medium (2 h St). Insets denote high magnification of the selected area. Scale bar, 5 μm. ( b ) Immuno-gold EM micrographs of HeLa cells transfected with GFP–PLD1 and subjected to 1 h of nutrient deprivation in the presence (St+B) or absence (St) of bafilomycin (50 nM). Insets denote high magnification of the selected area. Scale bar, 500 nm. Right panel: Histogram showing morphometric analysis of the relative distribution of GFP–PLD1-positive gold particles on the outer (arrows) and inner (arrowheads) membranes of the autophagosomal-like structures. Values denote means±s.e.m. ( n =14). ** P <0.01. Full size image PLD1 localizes to the outer membrane of amphisomes Immuno-EM analysis of nutrient-deprived HeLa cells with anti-GFP antibodies revealed gold particles for GFP–PLD1 on AP-like structures that exhibited a double membrane ( Fig. 1b ). Remarkably, the GFP–PLD1 immunoreactivity was predominantly ( ∼ 80%) found on the outer membrane of the AP-related structures after 1 h of nutrient deprivation. The gold particle distribution was insensitive to bafilomycin (that is, a blocker of lysosomal acidification), suggesting that the asymmetric distribution of GFP–PLD1 in AP-like structures is not accounted for by a selective degradation of GFP–PLD1 on the inner membrane. An alternate mechanism potentially underlying the enrichment of GFP–PLD1 on the outer membrane of AP-like structures is that PLD1 is translocated from endosomes to APs during the formation of amphisomes, a result of heterotypic fusion. If this is correct, there should be a pool of PLD1 co-localizing with both endosomal markers and LC3. Indeed, confocal analysis of nutrient-deprived HA–PLD1-transfected cells indicated that a significant fraction of anti-HA immunoreactivity was concomitantly positive for endogenous LC3 and various markers of the endosomal pathway, including Lamp1, Vps35, GFP–Rab5 and GFP–UVRAG ( Fig. 2 ). In contrast, no such co-localization was observed with Golgi marker giantin. 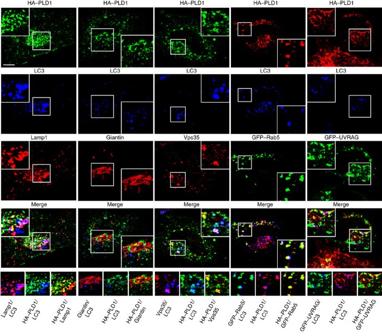Figure 2: PLD1 partially co-localizes with endogenous LC3 and endosomal markers upon nutrient deprivation. Confocal analysis of the subcellular localization of HA–PLD1 and endogenous LC3 using various organelle markers in cells deprived of nutrients for 2 h. Organelle markers used were as follows (from top to bottom panels): Lamp1 (late endosomes/lysosomes), giantin (Golgi-TGN), Vps35 (retromer-positive endosomes), GFP–Rab5 (early endosomes), GFP–UVRAG (early and late endosomes). Insets show high magnification of the selected areas. The triple insets at the bottom of each column of pictures indicate high magnification of the selected areas for two channels in various combinations. Scale bar, 5 μm. Figure 2: PLD1 partially co-localizes with endogenous LC3 and endosomal markers upon nutrient deprivation. Confocal analysis of the subcellular localization of HA–PLD1 and endogenous LC3 using various organelle markers in cells deprived of nutrients for 2 h. Organelle markers used were as follows (from top to bottom panels): Lamp1 (late endosomes/lysosomes), giantin (Golgi-TGN), Vps35 (retromer-positive endosomes), GFP–Rab5 (early endosomes), GFP–UVRAG (early and late endosomes). Insets show high magnification of the selected areas. The triple insets at the bottom of each column of pictures indicate high magnification of the selected areas for two channels in various combinations. Scale bar, 5 μm. Full size image Further supporting the idea that PLD1 is targeted to APs alongside endosomal membranes, HA–PLD1 was largely excluded from pre-autophagosomal structures based on the lack of co-localization with the markers ATG14L, GFP–ATG16L and ATG9 on nutrient deprivation for 2 h ( Fig. 3a and Supplementary Fig. S4 ). Additionally, a HeLa cell line stably expressing an inactive mutant version of Atg4B (Atg4BC74A), a protease that cleaves pro-LC3 paralogues, was used to investigate the localization of GFP–PLD1 on isolation membranes at the light microscopic ( Fig. 3b ) and ultrastructural levels ( Fig. 3c ). Atg4BC74A blocks the LC3-I to LC3-II conversion and causes defects in AP closure [22] , [23] . GFP–PLD1 did not co-localize with ATG16L in cells expressing Atg4BC74A ( Fig. 3b ), as expected from the fluorescent pattern of PLD1/ATG16L in wild-type (WT) HeLa cells ( Fig. 3a ). Furthermore, isolation membranes resulting from Atg4BC74A expression were virtually devoid of GFP immunoreactive gold particles ( Fig. 3c ), suggesting that GFP–PLD1 is transferred from endosomes to APs at a later stage in the autophagy process, that is, during amphisome formation. 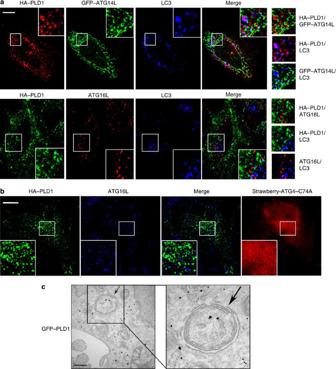Figure 3: PLD1 does not co-localize with markers of pre-autophagosomal structures and isolation membranes. (a) Confocal analysis of HeLa cells subjected to nutrient deprivation for 2 h. Cells were transfected with HA–PLD1 and GFP–ATG14L (upper panels) or with HA–PLD1 alone (lower panels). Upper panels: HA–PLD1 (red), GFP–ATG14L (green), endogenous LC3 (blue). Lower panels: HA–PLD1 (green), endogenous ATG16L (red) and LC3 (blue). Insets show high magnification of the selected areas. The triple insets on the right indicate high magnification of the selected areas for two channels in various combinations. Scale bar, 5 μm. (b) Confocal analysis showing lack of co-localization of HA–PLD1 (green) with the isolation membrane marker ATG16L (blue) in HeLa cells expressing the strawberry-ATG4–C74A mutant (red) and subjected to 1 h of nutrient deprivation. Insets denote high magnification of the selected area. Scale bar, 5 μm. (c) EM analysis showing that GFP–PLD1 does not localize to the isolation membrane (arrows) in cells expressing the strawberry-ATG4–C74A mutant. Immuno-gold EM micrographs of HeLa cells transfected with GFP–PLD1 and pStrawberry-ATG4–C74A and subjected to 1 h of nutrient deprivation. Inset denotes high magnification of the selected area. Scale bar, 250 nm. Figure 3: PLD1 does not co-localize with markers of pre-autophagosomal structures and isolation membranes. ( a ) Confocal analysis of HeLa cells subjected to nutrient deprivation for 2 h. Cells were transfected with HA–PLD1 and GFP–ATG14L (upper panels) or with HA–PLD1 alone (lower panels). Upper panels: HA–PLD1 (red), GFP–ATG14L (green), endogenous LC3 (blue). Lower panels: HA–PLD1 (green), endogenous ATG16L (red) and LC3 (blue). Insets show high magnification of the selected areas. The triple insets on the right indicate high magnification of the selected areas for two channels in various combinations. Scale bar, 5 μm. ( b ) Confocal analysis showing lack of co-localization of HA–PLD1 (green) with the isolation membrane marker ATG16L (blue) in HeLa cells expressing the strawberry-ATG4–C74A mutant (red) and subjected to 1 h of nutrient deprivation. Insets denote high magnification of the selected area. Scale bar, 5 μm. ( c ) EM analysis showing that GFP–PLD1 does not localize to the isolation membrane (arrows) in cells expressing the strawberry-ATG4–C74A mutant. Immuno-gold EM micrographs of HeLa cells transfected with GFP–PLD1 and pStrawberry-ATG4–C74A and subjected to 1 h of nutrient deprivation. Inset denotes high magnification of the selected area. Scale bar, 250 nm. Full size image Nutrient deprivation enhances PLD activity Next, the effect of nutrient deprivation on PLD activity was investigated. Total cellular PLD activity was measured by liquid chromatography–mass spectrometry analysis of its transphosphatidylation reaction product, phosphatidylethanol (PEtOH, Fig. 4a ), after incubation of cells with a low concentration of the primary alcohol ethanol [24] , [25] , [26] . An approximately twofold increase in PEtOH, a specific product of PLD, was found after 0.5-, 1.5- and 3-h nutrient deprivation ( Fig. 4a ). Other phospholipids, such as phosphatidylserine, phosphatidylethanolamine and PC, were not affected by starvation, whereas a trend for an increase in a variety of molecular species of PA was observed after 0.5 h starvation ( Supplementary Fig. S5a ). Treatment of cells with the PI-3 kinase inhibitor and autophagy blocker wortmannin [12] , [27] abolished the increase in PLD activity, suggesting that PLD1 lies downstream of a PI-3 kinase in the signalling cascade triggered by nutrient deprivation ( Fig. 4a ). 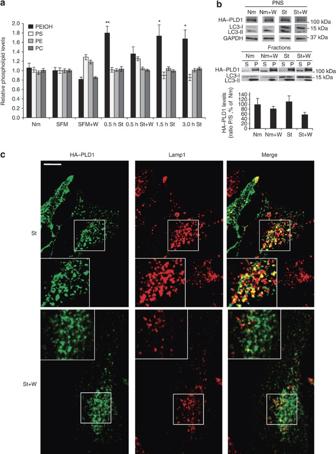Figure 4: The activity of PLD and subcellular localization of PLD1 are wortmannin sensitive. (a) Histogram showing relative phospholipid levels in CHO cells treated with 0.3% ethanol for 30 min before cell harvesting. Total PLD activity is measured as phosphatidylethanol (PEtOH) levels under the following conditions: normal medium (Nm), serum-free medium (SFM), serum-free medium with 100 nM wortmannin (SFM+W), nutrient deprivation (0.5 h St; 1.5 h St; 3.0 h St), 30 min of nutrient deprivation in presence of 100nM wortmannin (0.5h St+W). Other phospholipids were used as controls: phosphatidylserine (PS), phosphatidylethanolamine (PE), phosphatidylcholine (PC). Values denote means±s.e.m. (n=9, except for SFM+W and 0.5 h St+W, wheren=3 and 5, respectively). **P<0.01; *,P<0.05. (b) Western blot analysis of HA–PLD1 and endogenous LC3 levels in post-nuclear supernatant (PNS, upper panel), as well as in cytosolic/soluble (S) and particulate (P) fractions prepared from PNS after high-speed centrifugation (middle panel). GAPDH was used as loading control in PNS fractions. HeLa cells were transfected with expression vectors encoding HA–PLD1 for 24 h and subjected to 2 h of nutrient deprivation in the presence or absence of the PI3K inhibitor wortmannin (100 nM). Lower panel: quantitative analysis of HA–PLD1 immunoreactivity expressed as P/S ratio. Conditions were as follows: normal medium (Nm); normal medium with wortmannin (Nm+W); starvation condition (St); starvation condition+wortmannin (St+W). Values denote means±s.e.m. (n=3). (c) Confocal analysis of the co-localization between HA–PLD1 and Lamp1 in HeLa cells subjected to nutrient deprivation for 2 h in the presence (ST+W) or absence (St) of wortmannin 100 nM. Insets show high magnification of the selected areas. Scale bar, 5 μm. Figure 4: The activity of PLD and subcellular localization of PLD1 are wortmannin sensitive. ( a ) Histogram showing relative phospholipid levels in CHO cells treated with 0.3% ethanol for 30 min before cell harvesting. Total PLD activity is measured as phosphatidylethanol (PEtOH) levels under the following conditions: normal medium (Nm), serum-free medium (SFM), serum-free medium with 100 nM wortmannin (SFM+W), nutrient deprivation (0.5 h St; 1.5 h St; 3.0 h St), 30 min of nutrient deprivation in presence of 100nM wortmannin (0.5h St+W). Other phospholipids were used as controls: phosphatidylserine (PS), phosphatidylethanolamine (PE), phosphatidylcholine (PC). Values denote means±s.e.m. ( n =9, except for SFM+W and 0.5 h St+W, where n =3 and 5, respectively). ** P <0.01; *, P <0.05. ( b ) Western blot analysis of HA–PLD1 and endogenous LC3 levels in post-nuclear supernatant (PNS, upper panel), as well as in cytosolic/soluble (S) and particulate (P) fractions prepared from PNS after high-speed centrifugation (middle panel). GAPDH was used as loading control in PNS fractions. HeLa cells were transfected with expression vectors encoding HA–PLD1 for 24 h and subjected to 2 h of nutrient deprivation in the presence or absence of the PI3K inhibitor wortmannin (100 nM). Lower panel: quantitative analysis of HA–PLD1 immunoreactivity expressed as P/S ratio. Conditions were as follows: normal medium (Nm); normal medium with wortmannin (Nm+W); starvation condition (St); starvation condition+wortmannin (St+W). Values denote means±s.e.m. ( n =3). ( c ) Confocal analysis of the co-localization between HA–PLD1 and Lamp1 in HeLa cells subjected to nutrient deprivation for 2 h in the presence (ST+W) or absence (St) of wortmannin 100 nM. Insets show high magnification of the selected areas. Scale bar, 5 μm. Full size image Next, the effect of wortmannin was assessed on the membrane association of PLD1. Previous biochemical studies from others have shown that the majority of PLD1 is associated with membranes [28] . The association of PLD1 with membranes was first confirmed in HA–PLD1-transfected cells in normal medium using high-speed centrifugation and detection of anti-HA immunoreactivity predominantly in the particulate fraction with a minor pool found in the soluble (that is, cytosolic) fraction ( Fig. 4b ). As a control, LC3-II was exclusively found in the particulate fraction. Wortmannin treatment slightly enhanced the cytosolic pool of HA–PLD1 in normal medium ( Fig. 4b ). Importantly, the PI-3 kinase blocker more significantly decreased the membrane association (and correspondingly enhanced the cytosolic pool) of HA–PLD1 upon nutrient deprivation. Wortmannin also decreased the LC3-II/LC3-I ratio to 23.0±8.3% of control levels ( n =3; P <0.01) in the post-nuclear supernatant ( Fig. 4b ) and LC3-positive puncta formation as well ( Supplementary Fig. S5b ), indicating autophagy inhibition. Accordingly, the anti-HA signal was decreased in immunofluorescence and resulted in a loss of co-localization of HA–PLD1 with Lamp1 ( Fig. 4c ) and Vps35 ( Supplementary Fig. S5c ) in starved cells during treatment with wortmannin, but did not cause a redistribution of HA–PLD1 fluorescence into the Golgi ( Supplementary Fig. S5d ). Collectively, these data suggest that the subcellular localization of PLD1 during nutrient deprivation is controlled by a wortmannin-sensitive PI-3 kinase. Vps34 silencing and PX domain mutations affect PLD1 Class III PI-3 kinase Vps34 is believed to be a main target of wortmannin in the absence of nutrients and is a master regulator of autophagy [12] , [27] . Because the localization of PLD1 is sensitive to wortmannin, it is likely to depend on Vps34 and its NH 2 -terminal PI(3)P-binding PX module [29] , [30] . To test this, HeLa cells were treated with short interfering RNAs (siRNAs) against Vps34 (siVps34) or control siRNAs (siCtrl), followed by expression of HA–PLD1. Levels of Vps34 were decreased by ∼ 90% following siVps34 treatment ( Fig. 5a ). Silencing Vps34 decreased the LC3 fluorescence upon nutrient deprivation, consistent with a block in autophagy ( Fig. 5b ). Remarkably, the levels of HA–PLD1 were dramatically decreased on silencing of Vps34, based on both western blot and immunofluorescence analyses ( Fig. 5a,b ), suggesting that Vps34 may be required for the stability of PLD1. In contrast, the levels of a control protein, amyloid precursor protein (whose expression is also driven by the CMV promoter), were unchanged by siVps34. Importantly, siVps34 treatment also produced an ∼ 50% decrease in the levels of endogenous PLD1, as measured by western blot analysis (data not shown). 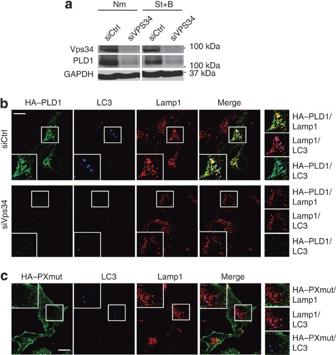Figure 5: The Vps34/PI(3)P pathway controls the expression levels and localization of PLD1. (a) Western blot analysis showing the effects of siRNA-mediated Vps34 (siVps34) downregulation on the expression levels of HA–PLD1 and Vps34 compared with control cells (siCtrl). Cells were incubated in normal medium (Nm) or subjected to 2 h of nutrient deprivation in the presence of 50 nM bafilomycin (St+B). HeLa cells were transfected for 48 h with siRNA directed to Vps34 (siVps34) or a control sequence (siCtrl) and then transfected for 24 h with a plasmid encoding HA–PLD1. (b) Confocal imaging showing the effects of Vps34 (siVps34) downregulation on HA–PLD1 (green), endogenous LC3 (blue) and Lamp1 (red) on 2 h of nutrient deprivation compared with control treatment (siCtrl). Scale bar, 5 μm. (c) Confocal analysis showing the subcellular localization of HA–PLD1 mutated in its PX domain (F120A/R179Q), so as to abolish phosphoinositide binding (HA–PXmut). HeLa cells were transiently transfected with a plasmid encoding HA–PXmut and fixed after 2 h of nutrient deprivation. HA–PXmut (green), endogenous LC3 (blue) and Lamp1 (red). Scale bar, 10 μm. Inbandc, insets show high magnification of the selected areas. The triple insets on the right indicate high magnification of the selected areas for two channels in various combinations. Figure 5: The Vps34/PI(3)P pathway controls the expression levels and localization of PLD1. ( a ) Western blot analysis showing the effects of siRNA-mediated Vps34 (siVps34) downregulation on the expression levels of HA–PLD1 and Vps34 compared with control cells (siCtrl). Cells were incubated in normal medium (Nm) or subjected to 2 h of nutrient deprivation in the presence of 50 nM bafilomycin (St+B). HeLa cells were transfected for 48 h with siRNA directed to Vps34 (siVps34) or a control sequence (siCtrl) and then transfected for 24 h with a plasmid encoding HA–PLD1. ( b ) Confocal imaging showing the effects of Vps34 (siVps34) downregulation on HA–PLD1 (green), endogenous LC3 (blue) and Lamp1 (red) on 2 h of nutrient deprivation compared with control treatment (siCtrl). Scale bar, 5 μm. ( c ) Confocal analysis showing the subcellular localization of HA–PLD1 mutated in its PX domain (F120A/R179Q), so as to abolish phosphoinositide binding (HA–PXmut). HeLa cells were transiently transfected with a plasmid encoding HA–PXmut and fixed after 2 h of nutrient deprivation. HA–PXmut (green), endogenous LC3 (blue) and Lamp1 (red). Scale bar, 10 μm. In b and c , insets show high magnification of the selected areas. The triple insets on the right indicate high magnification of the selected areas for two channels in various combinations. Full size image Next, a mutant version of HA–PLD1, harbouring mutations in the residues of the PX domain that mediates phosphoinositide binding (F120A/R179Q or PXmut) [29] , was expressed in HeLa cells. Unlike WT PLD1 ( Fig. 2 ), HA–PXmut was found mostly at the plasma membrane and did not co-localize with Lamp1 in normal media. It also failed to co-localize with Lamp1 and LC3 on starvation ( Fig. 5c ). The PX domain alone (amino acids 79–209) formed aggresomes (data not shown) and thus was not further investigated. Altogether, these data suggest that the proper subcellular localization of PLD1 in endosomes and AP-related structures is controlled by its PX domain and Vps34. However, because PI(3)P is present both on endosomes and on AP-related structures [8] , [46] , [47] , it is unclear whether binding of PX domain of PLD1 to this lipid on endosomes is sufficient to mediate the translocation of PLD1 from endosomes to APs during amphisome formation, or whether it needs to bind PI(3)P, both on endosomes and AP-related structures for this process to occur. Pharmacological inhibition of PLD decreases autophagy To explore the role of PLD1 in autophagy, primary alcohols were used as chemical inhibitors of the PLD pathway [17] . Cells were treated with 1-butanol or the control alcohol tert -butanol before confocal microscopic analysis. In normal media, the endogenous LC3 fluorescence was weak and diffuse as expected ( Supplementary Fig. S6a ). In contrast, nutrient starvation dramatically enhanced formation of discrete LC3-positive structures, both in number (fourfold) and total surface area (tenfold) ( Supplementary Fig. S6a,b ). Incubation with 1-butanol, but not with tert -butanol, reduced the number, the total surface area and the size of LC3-positive compartments ( Supplementary Fig. S6b ). Treatment with 1-butanol impaired LC3-II formation in both normal medium and after starvation ( Supplementary Fig. S6c ). Inhibition of lysosomal degradation, and thus AP clearance during starvation with bafilomycin caused LC3-II levels to dramatically increase ( Supplementary Fig. S6c ). This increase was much less pronounced in the presence of 1-butanol but not tert -butanol. Interestingly, 1-butanol also appeared to slightly decrease the levels of LC3-I in normal media. These results suggest that reducing PLD-mediated PA synthesis decreases the expansion of LC3-positive compartments. Next, a small molecule inhibitor of PLD, 5-fluoro-2-indolyl des-chlorohalopemide (FIPI) was used [31] . Confocal analysis of LC3-positive compartments in CHO cells following a 3-h nutrient starvation period revealed that FIPI reduced their number by 33±9% ( Fig. 6a,b ). FIPI also caused a small but significant decrease in the size of LC3-positive compartments and a more pronounced reduction in the total surface area of these compartments ( Fig. 6b ). Finally, FIPI decreased the levels of LC3-II in starvation and starvation + bafilomycin conditions ( Fig. 6c ). 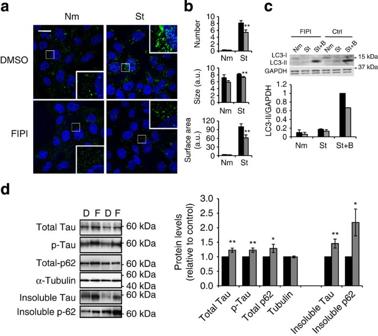Figure 6: FIPI reduces nutrient starvation-induced autophagy and the clearance of protein aggregates. (a) Confocal analysis showing the effects of PLD inhibition (FIPI, 750 nM) on the levels of endogenous LC3. CHO cells were treated with PLD inhibitor FIPI or DMSO for 3 h in the presence of serum (normal medium, Nm) or in the absence of nutrients (starvation, St). Insets denote high magnification of the selected areas. Scale bar, 10 μm. (b) Quantification of the average number, size and surface area of LC3-positive compartments per cell after FIPI treatment. Black bars, DMSO (vehicle); grey bars, FIPI treatment. Values denote means±s.e.m. (n=180–285 cells for Nm;n=449–519 cells for St). **P<0.01. (c) Western blot analysis showing levels of LC3-I and LC3-II in control- and FIPI-treated CHO cells grown in normal medium (Nm), after nutrient starvation (St) or after nutrient starvation in the presence of 50 nM bafilomycin (St+B). Treatments were for 3 h. Right panel: quantification of protein signal intensities showing LC3-II protein levels in extracts from nutrient-starved and bafilomycin-treated CHO cells following FIPI treatment. Black bars, DMSO (vehicle); grey bars, FIPI treatment. Values denote means±s.e.m. (n=4). (d) Western blot analysis of the effects of PLD inhibition on the levels of total Tau, phosphorylated Tau (p-Tau) and detergent-insoluble Tau. Organotypic brain slices from hTau mice were treated with either DMSO (D) or 750nM FIPI (F) and harvested after 5 days of treatment. Left panel: western blot analysis showing immunoreactivities for total human Tau (CP27), hyperphosphorylated tau (p-Tau, ser202/ser205, CP13), p62 and tubulin from the supernatant fraction and aggregated tau (CP27) and p62 from the sarkosyl-insoluble fraction. Two representative pairs are displayed. Right panel, quantification of total proteins (Tau, p-Tau, p62 and tubulin) and sarkosyl-insoluble aggregates of tau (insoluble Tau) and p62 (insoluble p62). Black bars, DMSO (vehicle); grey bars, FIPI treatment. Values denote means±s.e.m. (n=7). **P<0.01; *,P<0.05. For the statistical analysis of FIPI-treated samples, tau and p62 protein levels were compared with tubulin. Figure 6: FIPI reduces nutrient starvation-induced autophagy and the clearance of protein aggregates. ( a ) Confocal analysis showing the effects of PLD inhibition (FIPI, 750 nM) on the levels of endogenous LC3. CHO cells were treated with PLD inhibitor FIPI or DMSO for 3 h in the presence of serum (normal medium, Nm) or in the absence of nutrients (starvation, St). Insets denote high magnification of the selected areas. Scale bar, 10 μm. ( b ) Quantification of the average number, size and surface area of LC3-positive compartments per cell after FIPI treatment. Black bars, DMSO (vehicle); grey bars, FIPI treatment. Values denote means±s.e.m. ( n =180–285 cells for Nm; n =449–519 cells for St). ** P <0.01. ( c ) Western blot analysis showing levels of LC3-I and LC3-II in control- and FIPI-treated CHO cells grown in normal medium (Nm), after nutrient starvation (St) or after nutrient starvation in the presence of 50 nM bafilomycin (St+B). Treatments were for 3 h. Right panel: quantification of protein signal intensities showing LC3-II protein levels in extracts from nutrient-starved and bafilomycin-treated CHO cells following FIPI treatment. Black bars, DMSO (vehicle); grey bars, FIPI treatment. Values denote means±s.e.m. ( n =4). ( d ) Western blot analysis of the effects of PLD inhibition on the levels of total Tau, phosphorylated Tau (p-Tau) and detergent-insoluble Tau. Organotypic brain slices from hTau mice were treated with either DMSO (D) or 750nM FIPI (F) and harvested after 5 days of treatment. Left panel: western blot analysis showing immunoreactivities for total human Tau (CP27), hyperphosphorylated tau (p-Tau, ser202/ser205, CP13), p62 and tubulin from the supernatant fraction and aggregated tau (CP27) and p62 from the sarkosyl-insoluble fraction. Two representative pairs are displayed. Right panel, quantification of total proteins (Tau, p-Tau, p62 and tubulin) and sarkosyl-insoluble aggregates of tau (insoluble Tau) and p62 (insoluble p62). Black bars, DMSO (vehicle); grey bars, FIPI treatment. Values denote means±s.e.m. ( n =7). ** P <0.01; *, P <0.05. For the statistical analysis of FIPI-treated samples, tau and p62 protein levels were compared with tubulin. Full size image Blockade of PLD leads to aggregate accumulation FIPI was further explored for its ability to impair autophagy-mediated clearance of protein aggregates in an ex vivo model of tauopathy, in which the microtubule-binding protein Tau accumulates in the form of insoluble hyperphosphorylated aggregates [32] , [33] . Briefly, brain slices derived from a transgenic mouse overexpressing human WT Tau in a murine Tau knockout (KO) background were treated for 5 days, either with FIPI or vehicle (dimethylsulphoxide, DMSO). After the treatment, total protein extracts and sarcosyl-insoluble Tau were analysed by immunoblotting ( Fig. 6d ). Although FIPI had a subtle effect on the levels of total Tau and phosphorylated Tau (that is, an ∼ 20% increase), it has a more pronounced effect on detergent-insoluble Tau (that is, an ∼ 50% increase; Fig. 6d ). p62, a protein that is predominantly degraded by autophagy, showed a similar pattern, although the impact of FIPI on insoluble p62 was more evident (that is, an ∼ 2.2-fold increase). Collectively, these results suggest that the catalytic activity of PLD regulates the clearance of protein aggregates, consistent with a role in autophagy (although a role for PLD in regulating other aspects of Tau metabolism cannot be excluded). PLD1-deficient fibroblasts exhibit autophagy defects As part of our original screen, we used RNA interference against PLD1 to validate the involvement of this gene in autophagy. Expression of short hairpin RNAs (shRNA) to PLD1 (shPLD1) significantly decreased the protein levels of PLD1 and the number of autophagic cells during starvation relative to control shRNA ( Supplementary Fig. S7a,b ). EM analysis of starved HeLa cells revealed a dramatic decrease in the number of APs after silencing of PLD1, consistent with the fluorescence microscopy data ( Supplementary Fig. S7c ). To expand this analysis and genetically test for the involvement of PLD1 in autophagy, mice lacking PLD1 were engineered using homologous recombination ( Supplementary Fig. S8a–d ). Pld1 KO animals develop normally and reach adulthood indistinguishably from WT mice, as previously observed by others [34] . Fibroblasts were derived from WT and KO embryos, immortalized and tested for a potential autophagy defect after verification of PLD1 ablation ( Supplementary Fig. S8e ). Western blot analysis showed reduced levels of LC3-II in nutrient-deprived Pld1 KO MEFs (mouse embryonic fibroblasts) in the presence or absence of bafilomycin ( Fig. 7a,b ). Interestingly, the levels of LC3-I also appeared to decrease in KO MEFs ( Fig. 7a ), although this phenomenon was not observed in KO liver tissue ( Supplementary Fig. S8f ). Confocal microscopic analysis of endogenous LC3 showed consistent results, with a lesser number and smaller size of LC3-positive structures in Pld1 KO MEFs ( Fig. 7c,d ). Thus, MEFs lacking PLD1 exhibit defects in starvation-induced autophagy. 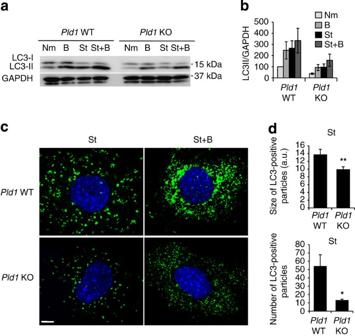Figure 7: Ablation of PLD1 in MEFs produces a defect in starvation-induced autophagy. (a) Western blot analysis showing reduced levels of LC3-II in KO MEFs. (b) Quantification of protein signal intensities from western blots showing LC3-II levels in MEFs extracts after normalization to the control protein GAPDH. Inaandb, MEFs were grown in normal medium (Nm), treated for 2 h with 50 nM bafilomycin in normal medium (B), or grown in nutrient-deprived medium in the absence (St) or presence of 50 nM bafilomycin (St+B). Values denote means±s.e.m. (n=4). (c) Immunostaining of endogenous LC3 inPld1WT and KO MEFs showing a reduced number and size of the LC3-positive compartment in KO MEFs. The DAPI staining is shown in blue. Cells were deprived of nutrients for 2 h in the absence (St, upper panels) or presence of bafilomycin (St+B, lower panels). Scale bar, 5 μm. (d) Quantification of the average size (top panel) and number of LC3-positive compartments per cell (bottom panel) inPld1WT and KO MEFs starved for 2 h. Values denote means±s.e.m. (n=6, number of cells=26–45 for all the conditions). **P<0.01; *P<0.05. Figure 7: Ablation of PLD1 in MEFs produces a defect in starvation-induced autophagy. ( a ) Western blot analysis showing reduced levels of LC3-II in KO MEFs. ( b ) Quantification of protein signal intensities from western blots showing LC3-II levels in MEFs extracts after normalization to the control protein GAPDH. In a and b , MEFs were grown in normal medium (Nm), treated for 2 h with 50 nM bafilomycin in normal medium (B), or grown in nutrient-deprived medium in the absence (St) or presence of 50 nM bafilomycin (St+B). Values denote means±s.e.m. ( n =4). ( c ) Immunostaining of endogenous LC3 in Pld1 WT and KO MEFs showing a reduced number and size of the LC3-positive compartment in KO MEFs. The DAPI staining is shown in blue. Cells were deprived of nutrients for 2 h in the absence (St, upper panels) or presence of bafilomycin (St+B, lower panels). Scale bar, 5 μm. ( d ) Quantification of the average size (top panel) and number of LC3-positive compartments per cell (bottom panel) in Pld1 WT and KO MEFs starved for 2 h. Values denote means±s.e.m. ( n =6, number of cells=26–45 for all the conditions). ** P <0.01; * P <0.05. Full size image PLD1 ablation results in autophagy defects in the liver To test whether PLD1 is involved in autophagy in vivo , liver from WT and KO mice was analysed, as this tissue is associated with extensive autophagic activity. Immunofluorescence analysis of liver tissue sections using anti-LC3 antibodies revealed that nutrient starvation for 24 h in WT mice significantly increased the average size as well as the surface area (per field) of the LC3-positive compartment, with a lesser effect on the compartment number ( Fig. 8a,b ). In contrast, food restriction failed to expand the LC3-positive compartment in KO liver ( Fig. 8a,b ). Light microscopic observations were corroborated by EM analysis, which showed an increase in both the average number and surface area of APs/amphisomes after 24-h starvation in WT, but not in KO sections ( Fig. 8c,d ). Comparable results were obtained with autophagolysosomes/lysosomes. Interestingly, morphometric analysis showed that APs, but not autophagolysosomes/lysosomes, are smaller in KO liver ( Fig. 8e ). Consistent with the microscopy, western blot analysis showed that LC3-II levels fail to increase after food restriction in KO liver ( Supplementary Fig. 8f ). Finally, to exclude possible defects in autophagy due to differences in food intake or in metabolism, blood glucose and insulin levels were measured in normally fed and starved mice, and no differences were found between genotypes ( Supplementary Fig. S9 ). In conclusion, these findings provide in vivo and genetic evidence for the involvement of PLD1 in the regulation of starvation-induced autophagy in the liver. 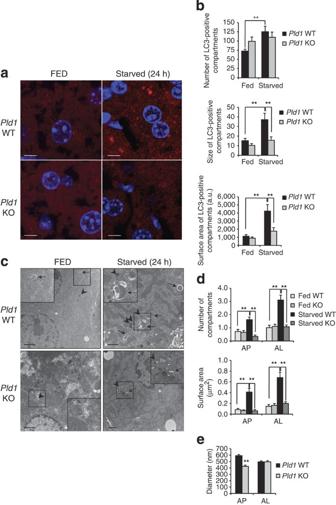Figure 8: Morphological analysis showing reduced hepatic autophagy in starved PLD1-deficient mice. (a) Immunofluorescent detection of endogenous LC3 (red) in liver sections from fed or starvedPld1WT and KO mice. Sections were counterstained with DAPI. Scale bar, 5 μm. (b) Quantitative analysis of endogenous LC3 immunofluorescence in liver sections derived from fed or starvedPld1WT and KO mice. Histograms show the average number, size and surface area of LC3-positive compartments. Values denote means±s.e.m. ((n=25–28), 4 mice per genotype). **P<0.01. (c) Electron microscopic analysis showing a reduction in the size and number of autophagosome/amphisome-like structures (AP) in PLD1-deficient mice after food restriction. Representative electron micrographs from animals analysed inashowing APs (arrows) and autophagolysosomes/lysosomes (AL, arrowheads) in liver sections from starved WT and KO mice. Insets show high magnification of the selected areas. Scale bar, 1 μm. (d) Morphometric analysis of the number (per 100 μm2cytoplasmic area) and relative surface area (% cytoplasmic area) of APs and ALs. Values denote means±s.e.m. (n=36 electron micrograms, from a total of 3,600 μm2cytoplasmic area per genotype). **P<0.01. (c) Morphometric analysis of the diameter of APs and ALs in the liver of PLD1-deficient mice after food restriction. Values denote means±s.e.m. (n=60). **P<0.01. Figure 8: Morphological analysis showing reduced hepatic autophagy in starved PLD1-deficient mice. ( a ) Immunofluorescent detection of endogenous LC3 (red) in liver sections from fed or starved Pld1 WT and KO mice. Sections were counterstained with DAPI. Scale bar, 5 μm. ( b ) Quantitative analysis of endogenous LC3 immunofluorescence in liver sections derived from fed or starved Pld1 WT and KO mice. Histograms show the average number, size and surface area of LC3-positive compartments. Values denote means±s.e.m. (( n =25–28), 4 mice per genotype). ** P <0.01. ( c ) Electron microscopic analysis showing a reduction in the size and number of autophagosome/amphisome-like structures (AP) in PLD1-deficient mice after food restriction. Representative electron micrographs from animals analysed in a showing APs (arrows) and autophagolysosomes/lysosomes (AL, arrowheads) in liver sections from starved WT and KO mice. Insets show high magnification of the selected areas. Scale bar, 1 μm. ( d ) Morphometric analysis of the number (per 100 μm 2 cytoplasmic area) and relative surface area (% cytoplasmic area) of APs and ALs. Values denote means±s.e.m. ( n =36 electron micrograms, from a total of 3,600 μm 2 cytoplasmic area per genotype). ** P <0.01. ( c ) Morphometric analysis of the diameter of APs and ALs in the liver of PLD1-deficient mice after food restriction. Values denote means±s.e.m. ( n =60). ** P <0.01. Full size image Collectively, results from our study demonstrate that PLD1 localizes to AP-related organelles and primarily regulates their maturation step in the autophagy process, likely as a downstream effector of Vps34. Although the majority of our data point to a role of PLD1 in starvation-induced autophagy, results from pharmacological blockade experiments suggest that its function may also be relevant for the autophagy-mediated clearance of protein aggregates, such as those consisting of p62 and Tau, with potentially major implications for a variety of neurodegenerative disorders, including tauopathies. Altogether, this study introduces a PLD1 as a new player in the molecular machinery governing autophagy. Consistent with the physicochemical properties of its product PA (that is, a cone-shaped lipid), PLD1 has been previously shown to have pleiotropic roles linked to membrane trafficking [17] , [18] , [35] . In particular, several reports point to a role of PLD1 in the fusion of various secretory organelles with the plasma membrane [35] , [36] , [37] , [38] , [39] , [40] , although genetic evidence in support of such findings is lacking. There is however strong genetic evidence connecting the yeast PLD orthologue, Spo14, to membrane fusion and, more specifically, to the formation of prospore membranes during meiosis [20] . More recent evidence has implicated Spo14 in unconventional secretion of Pichia pastoris Acb1, a process also depending on AP formation and their fusion with the plasma membrane [21] . Although yeast PLD does not appear to be required for canonical autophagy (ref. 21 ; R. Manjithava and S. Subramani, personal communication), work on this organism implicates this enzyme in the fusion of intracellular organelles in response to stress; thus, suggesting an interesting analogy with the expansion of APs in response to nutrient deprivation. Our study strongly suggests that mammalian PLD1 facilitates the maturation of APs during starvation-induced autophagy. Indeed, we find that PLD1 is predominantly associated with endosomes in normal medium and that a pool of this enzyme translocates onto LC3-positive structures upon nutrient deprivation. Because these compartments are also positive for endosomal markers, we speculate that they may originate from the heterotypic fusion of endosomes with APs and thus correspond to bona fide amphisomes, as seen in other instances [7] , [41] , [42] , [43] , [44] . EM analysis provided strong support to this hypothesis, as the immunoreactivity of PLD1 predominantly localized to the outer membrane of AP-related structures, suggesting that the asymmetric distribution of PLD1 may simply reflect its redistribution from the limiting membrane of endosomes to the outer membrane of amphisomes following fusion of endosomes with APs. Although the mere translocation of PLD1 from endosomes to amphisomes does not prove an implication of this lipid enzyme in the maturation of APs, our functional analyses indicate that interfering with the function of PLD1 significantly alters the metabolism of LC3-II, as well as the size and number of APs, thus pointing to a relevant role of this enzyme in autophagy. Although these phenotypes are, in principle, also consistent with an involvement of PLD1 in the biogenesis of APs, they cannot be easily reconciled with the fact that PLD1 is absent from isolation membranes in cells expressing the Atg4C mutant. However, it is of note that regulation of AP biogenesis from an ' in-trans' location of PLD1 cannot be excluded (for example, PLD1 may hydrolyse PC on pre-autophagosomal membranes while residing on endosomes). Collectively, our results implicate PLD1 in the maturation step, as well as suggest a possible role for this lipid enzyme in the biogenesis of APs. Although 1-butanol and FIPI are not specific inhibitors of the PLD1 pathway, their deleterious effects on autophagy indicates that the catalytic activity of PLD, and thus PA formation, is required for this action. Accordingly, total PLD activity is stimulated by nutrient starvation. We speculate that elevation of PA on AP/endosomal membranes may facilitate their fusion and thus the formation of amphisomes. However, we were only able to detect a very small pool of PA on AP membranes using immuno-EM analysis of GFP–Spo20, a genetically encoded probe for PA (data not shown). This is indicative of either a transient role for this lipid in the PLD1 pathway and/or a rapid conversion of PA into downstream metabolites, such as diacylglycerol, on APs/amphisomes. Interestingly, a recent study showed that a pool of diacylglycerol produced by PA phosphatases downstream of PLD is a signal required for the initiation of Salmonella -induced autophagy [45] . Finally, in addition to changing the physicochemical properties of membrane bilayers, PA has an important signalling role and may exert its actions through effectors, such as mTOR [19] , [49] , [50] . Although activation of mTOR suppresses autophagy [51] , PLD1 may function as both positive and negative modulator of the mTOR pathway, depending on its subcellular localization, the cell state and the experimental conditions. Such a dual role has been previously described for Vps34, a lipid enzyme that is required for autophagy, yet also stimulates mTOR [12] , [51] . Although the precise role of PA in autophagy remains to be elucidated, the upstream regulation of PLD1 in the autophagy pathway has begun to be unravelled and likely involves the class III PI-3 kinase Vps34 and its product PI(3)P [8] , [12] . One of the first requirements during autophagy activation is the synthesis of PI(3)P by Vps34, which control both the biogenesis and maturation of APs [8] , [46] , [47] in addition to being a master regulator of the endosomal pathway [13] . Interestingly, sensory neuron-specific ablation of Vps34 produces defects in the endolysosomal pathway and neurodegeneration, although a non-canonical type of autophagy may occur in mutant neurons [48] . Our study suggests that PLD1 may be an effector of the Vps34/PI(3)P pathway modulating AP maturation, based on experiments involving wortmannin, Vps34 silencing and the PX mutant of PLD1 that is deficient in phosphoinositide binding. Future work will address the exact nature of the Vps34 subcomplexes [8] and the lipid-based targeting mechanism controlling the function of PLD1 in autophagy. In particular, it will be important to determine whether the translocation of PLD1 from endosomes to APs during the maturation process requires an interaction of its PX domain with a pool of PI(3)P (and potentially other D3-phosphoinositides) located on endosomes, on AP-related structures themselves or on both these organelles. In summary, our findings demonstrate a novel role for PLD1 in the regulation of autophagy and, in particular, in the maturation of APs as a possible effector downstream of the Vps34/PI(3)P pathway. Because the ablation of PLD1 does not produce any overt anomalies in the mouse (this study; also see ref. 34 ), unlike ablation of core components of the autophagy machinery [52] , [53] , we speculate that PLD1 ablation may spare basal autophagy and primarily target starvation-induced autophagy. However, the FIPI experiments showing that blocking PLD may delay the clearance of protein aggregates suggest an involvement of PLD1 in pathways other than starvation-induced autophagy. Despite these considerations, blocking the PLD1 pathway may be a suitable approach for potential therapeutic interventions in specific disorders, whereby autophagy inhibition may be beneficial, such as cancer and ischaemia. Importantly, our recent studies have shown that the ablation of PLD2 confers protection against the synaptotoxic effects of β-amyloid in neuronal cultures and in a mouse model of Alzheimer's disease [54] , [55] . Thus, targeting PLD isozymes with small molecules may be beneficial in a growing number of human disorders. In this respect, the recent development of isoform-specific inhibitors may prove helpful [56] . Molecular biology and antibodies The information regarding molecular biology and antibodies can be found in Supplementary methods . Cell culture and transfection HeLa (human cervical cancer) cells and MEFs (murine embryonic fibroblast) were grown at 37 °C in a 5% CO 2 incubator in DMEM (Invitrogen). CHO (Chinese Hamster Ovary) were grown in F12 medium. HeLa cells were transiently transfected with the Lipofectamine 2000 reagent (Invitrogen) using the manufacturer's instructions. Detailed information can be found in Supplementary methods . Pld1 knockout mice and MEFs Pld1 Flox Neo/+ mice were bred with Rosa26 Cre/Cre mice, which express Cre recombinase, to eliminate exons 13 and 14 and produce Pld1 +/− mice. Pld1 +/− mice were then intercrossed to create Pld1 +/+ and Pld1 −/− mice. Ablation of PLD1 was monitored by PCR and immunoblotting (see Supplementary methods ). In some experiments, animals were starved for 24 h to induce autophagy. For the metabolic studies see Supplementary methods . Pld1 +/+ and Pld1 −/− mice were used to isolate MEFs (13.5-day embryos; see Supplementary methods ). Cell were plated in a 100 mm dish and labelled as passage 0. Each culture was derived from a single embryo and 1.2 × 10 6 cells per dish were subsequently plated and passaged every 3–4 days. MEFs were used after immortalization (around passage 25). All experiments involving animals were made in accordance with protocols approved by the Institutional Animal Care and Use Committee of Columbia University. Lipid analysis CHO cells cultured in 100 mm plates were incubated for 3 h in serum-free medium or subjected to a time course in Hank's balanced salt solution (HBSS) for 0.5, 1.5 and 3 h in order to promote starvation-induced autophagy. For PLD activity measurement, 0.3% ethanol (in the presence or absence of 100 nM wortmannin) was added to the medium 30 min before harvesting the cells. Cells were then resuspended in a solution of methanol and chloroform (2:1), vortexed for 1 min and incubated on ice for 5 min. These last two steps were repeated three times. For lipid extraction KCl (1 M; 1:10 volume) was added to the lysates and samples were centrifuged for 2 min at 7,500× g at 4 °C. The organic phase was recovered and extracted lipids were dried and stored at −80 °C. Lipid extracts were spiked with internal standards and analysed by liquid chromatography–mass spectrometry using multiple reactions monitoring (see Supplementary methods ). Subcellular fractionation HeLa cells were transiently transfected with a construct encoding HA–PLD1 for 24 h. Cells in confluent monolayers were kept growing in normal medium or starved in HBSS in the presence or absence of wortmannin (100 nM) for 2 h. Media containing wortmannin were replaced every 45 min. Following the treatments, cells were scraped in 3 ml of cold PBS and centrifuged for 5 min at 100× g at 4 °C. After rinsing the cells in 3 ml of homogenization buffer (HB: 8% sucrose in PBS), cell pellets were centrifuged for 10 min at 400× g at 4 °C. Cells were then resuspended in 0.2 ml of HB and harvested by three passages through a 22-G 1¼ needle on a 1-ml plastic syringe. Homogenates were centrifuged for 10 min at 400× g at 4 °C, and post-nuclear supernatants were collected. Cytosol and membranes were prepared by centrifugation of the supernatants at 200,000× g at 4 °C for 30 min. Pellets were then resuspended in the same volume of HB as the cytosol fraction. Samples were separated on an SDS–polyacrylamide gel electrophoresis (PAGE; 8–16%) and analysed by immunoblotting. Alcohol and FIPI treatments CHO or HeLa cells were treated with 0.3% alcohol (ethanol, 1-butanol or tert -butanol) for 3 h, either in normal medium or in HBSS. In some experiments, cells were pre-treated with FIPI (750 nM) or DMSO (vehicle), before nutrient deprivation. Cells were then processed for western blotting or immunofluorescence analysis. To assess the effect of FIPI on the levels of Tau and p62 aggregates, organotypic brain slices from transgenic mice overexpressing human Tau in the mouse Tau KO background were used [32] , [33] . Sarcosyl-insoluble material was analysed by SDS–PAGE and immunoblotting (see Supplementary methods ). Western blotting and detection of endogenous LC3 CHO or HeLa cells plated in 100-mm dishes were lysed in 300 μl of lysis buffer (50 mM Tris–HCl (pH 7.2), 250 mM NaCl, 0.1% NP-40, 2 mM EDTA, 10% glycerol). Extracts were then centrifuged at 16,000× g for 30 min at 4 °C, before protein quantification using the Coomassie Plus-200 protein assay reagent (Pierce). Proteins in SDS sample buffer were separated by SDS–PAGE and transferred onto polyvinylidene difluoride membranes. Membranes were probed with the indicated primary antibodies. Secondary antibodies were conjugated with horseradish peroxidase or with infrared (IR)-dyes for IR signal detection. For IR, membranes were exposed and analysed on the Odyssey Infrared Imaging System (LI-COR Biosciences) and the Odyssey software; for horseradish peroxidase, images were and captured using a Fuji LAS4000 Imaging unit (GE Healthcare) and analysed using ImageJ software (NIH). Immunofluorescence on cultured cells CHO or HeLa cells were grown on coverslips (confluence ∼ 70%). After treatments, cells were washed three times with ice-cold PBS, fixed with 4% paraformaldehyde for 20 min at room temperature (RT) and washed three times with PBS. They were then permeabilized with 200 μg ml −1 digitonin (Invitrogen) for 15 min and incubated for 1 h at RT with primary antibodies diluted in PBS. After three washes with PBS, cells were incubated with Alexa Fluor or Cy3-conjugated secondary antibodies for 1 h at RT, washed three times in PBS and coverslips were mounted in Vectashield with DAPI (Vector). Images were acquired by confocal microscopy (Zeiss LSM-700 (Zeiss) or Nikon EZ-C1.2.30 (Nikon)). Immunofluorescence on tissue sections Mouse livers were cut in small pieces before immersion fixation in 4% paraformaldehyde for 18 h at 4 °C. For the post-fixation, specimens were immersed in 15% sucrose solution for 4 h at RT and transferred to a 30% sucrose solution for 24 h at 4°C. Immunohistochemistry was performed on 5-μm-thick slices obtained with a cryostat. A blocking step was performed using 5% donkey serum in PBS for 30 min, before staining with an anti-LC3 antibody (Novus) for 1 h at RT. After three washes in PBS, specimens were incubated for 1 h with Alexa-555-conjugated secondary antibodies, rinsed three times in PBS and mounted using Vectashield medium containing DAPI (Vector). Images were acquired by confocal microscopy (Nikon EZ-C1.2.30, Nikon). Confocal microscopy and image analysis For the initial screen, HeLa cells transfected with GFP–PLD1 or shPLD1/shDsRED constructs alongside mRFP–LC3 constructs, were analysed using confocal z -stack images taken with the EZ-C1.3.0 acquisition software (Nikon EZ-C1.2.30, Nikon). Co-localization analysis was performed using the ImageJ software (NIH). For each field, the percent co-localization of green and red fluorescence was calculated as the ratio between the surface area of the single channel and the surface area matching both channels. For each experiment, 20 cells were analysed. Quantification of autophagic cells was performed as follows: cells were scored as 'autophagic' when the mRFP-LC3 fluorescence appeared as 20 or more punctate cytoplasmic structures (total number of cells counted=100–325). For the quantification of LC3-positive particles after alcohol and FIPI treatments, as well as in MEFs and liver slices, images were captured using confocal z -stack images taken with the EZ-C1.3.0 software (Nikon). Analysis was performed using the ImageJ software (NIH). LC3-positive compartments with a surface area of 4 pixels were automatically quantified for each field after subtraction of the background level. The number of LC3-positive compartments, the size (in pixel) and their surface areas (expressed as number of pixels per field) were normalized to the number of cells in each field. An average of 150 cells were analysed for each condition. For triple stainings, image acquisition was performed with a Zeiss LSM-700 confocal microscope and images were analysed using the ZEN software (Zeiss). EM analysis The pre-embedding gold enhancement immuno-gold method was used for the immuno-EM as described previously [57] with minor modifications. Standard fixation and embedding procedures were used for the processing of cell and tissue specimens (see supplementary methods for more details). Statistics At least three independent experiments were performed, unless indicated otherwise, in the figure legends. Statistical analyses were performed using two-tailed equal variance Student's t -test or one-way analysis of variance. P -values <0.05 and <0.01 were determined to be statistically significant (*) and highly significant (**), respectively. How to cite this article: Dall'Armi, C. et al . The phospholipase D1 pathway modulates macroautophagy. Nat. Commun. 1:142 doi: 10.1038/ncomms1144 (2010).